A chromatin activity-based chemoproteomic approach reveals a transcriptional repressome for gene-specific silencing Immune cells develop endotoxin tolerance (ET) after prolonged stimulation. ET increases the level of a repression mark H3K9me2 in the transcriptionally silent chromatin specifically associated with pro-inflammatory genes. However, it is not clear what proteins are functionally involved in this process. Here we show that a novel chromatin activity-based chemoproteomic (ChaC) approach can dissect the functional chromatin protein complexes that regulate ET-associated inflammation. Using UNC0638 that binds the enzymatically active H3K9-specific methyltransferase G9a/GLP, ChaC reveals that G9a is constitutively active at a G9a-dependent mega-dalton repressome in primary endotoxin-tolerant macrophages. G9a/GLP broadly impacts the ET-specific reprogramming of the histone code landscape, chromatin remodelling and the activities of select transcription factors. We discover that the G9a-dependent epigenetic environment promotes the transcriptional repression activity of c-Myc for gene-specific co-regulation of chronic inflammation. ChaC may also be applicable to dissect other functional protein complexes in the context of phenotypic chromatin architectures. Activation of inflammation is the key host response to microbial challenge, yet excessive production of pro-inflammatory cytokines can lead to tissue/organ damage or autoimmune diseases [1] , [2] . To minimize harmful effects caused by the continual presence of environmental stimuli, pre-exposed cells suppress cytokine production to become transiently unresponsive. However, this acquired immune tolerance is a double-edged sword, both protecting the host from infection/damage and, when dysregulated, contributing directly to various inflammation-associated pathologies [3] . Development of tolerance to endotoxin or lipopolysaccharide (LPS) is a major molecular feature of the pathogenesis of many chronic diseases including asthma, sepsis and cancer, as people experiencing endotoxin tolerance (ET) are immuno-compromised [4] , [5] . Recent studies have revealed that the control of inflammation is achieved primarily epigenetically in a gene-specific manner, whereby, with prolonged LPS stimulation, chromatin associated with pro-inflammatory or ‘tolerizeable’ genes (T-genes) becomes transcriptionally silenced [6] , [7] . Unknown, however, are the functional constituents of the inflammation-phenotype chromatin architecture that directly participate in transcription regulation of select genes. Histone post-translational modifications (PTMs), such as acetylation, phosphorylation and methylation, determine the functional state of chromatin, which eventually controls chromatin-mediated transcription [8] . Meanwhile, the levels of particular histone PTM(s) are regulated by corresponding histone-modifying enzymes, whose activities vary under different cell states [9] . Specifically, within transcriptionally silenced chromatin, dimethylated lysine 9 on histone H3 (H3K9me2), a code for transcriptional repression, is higher in abundance compared to the transcriptionally active chromatin of LPS-responsive cells [10] , implicating that the H3K9me2 writer, a histone methyltransferase (HMTase) G9a (refs 11 , 12 ) is more enzymatically active in LPS-tolerant macrophages. Further, G9a was identified as a common component of different protein co-repressor complexes [13] , [14] , [15] , [16] and was also found to interact with various chromatin effectors [17] . In addition, a growing number of non-histone substrates of G9a have been identified [18] . These data led us to hypothesize that within transcriptionally silenced chromatin, G9 exercises a wide spread function in gene-specific transcriptional regulation by coordinating a chromatin writer assembly involving multiple, distinct protein complexes (or ‘complexome’) [19] . Emerging activity-based protein profiling (ABPP) strategies provide a functional assessment of particular classes of proteins/enzymes including kinases, proteases, phosphatases, glycosidases and oxidoreductases in defined cell states [20] . Further, quantitative ABPP allows comparison of the target phenotypic activities with identification of their activity-based complex companions in cells [21] . While the emergence of newly synthesized chemicals that show high specificity in recognizing different histone-modifying enzymes enables the proteome-wide analysis of their activities in various live cells [22] , [23] , [24] , [25] , the unique strength of emerging chemoprobes of corresponding histone-modifying enzymes needs to be explored to dissect various epigenetic protein machinery operating under defined phenotypic cell states. Here we use UNC0638 (ref. 26 ), a substrate-competitive inhibitor/chemoprobe that selectively binds enzymatically active G9a, to design a novel chromatin activity-based chemoproteomic (ChaC) approach to systematically characterize proteins specifically complexed with the phenotypically active G9a within the gene-specific chromatin of defined transcriptional states. Proteins (606) are identified to have enhanced interactions with activated G9a within ET-characteristic chromatin, while their associations with G9a are weakened or undetectable in acute-inflamed macrophages. This inflammation-phenotype ChaC analysis indicates that chronically active G9a promotes assembly of an ET-characteristic complexome. Further characterization of our function-based ChaC proteomic findings reveals that chronically active G9a not only coordinates the deposition of combinatorial methyl-lysine codes on H3 but also stabilizes select transcription factors in cross talk to promote their co-repression of select genes. Specifically, we discover a new G9a-dependent role of c-Myc in regulating select genes under chronic inflammation, whereby chronically active G9a directs c-Myc toward a transcription repressor by stabilizing c-Myc within a gene-specific, methyl-lysine-rich chromatin environment. On a systems view within the chromatin associated with specific genes, chronically active G9a/GLP preserves the integrity of the protein complexes for ET-characteristic transcriptional repression, a protein ‘repressome’ [27] . ChaC methodology reveals how this repressome complex is built, localized, and regulated in a gene-specific manner. Histone H3 PTM is reprogrammed in ET macrophages To determine exactly how histone H3 is differentially modified during the macrophage response to acute versus chronic LPS stimulation, we first used top–down MS [28] to map the PTM landscape of full-length H3 from bone marrow-derived macrophages (BMDMs) under the following inflammatory states [7] : non-stimulated (naïve or ‘N’) cells, cells stimulated with a single high-dose LPS (LPS-responsive or ‘NL’), cells primed with a low-dose LPS (LPS-tolerant or ‘T’) and LPS-tolerant cells restimulated with a high-dose LPS that mimics ET (‘TL’; Supplementary Fig. 1a ). Following histone extraction and high-performance liquid chromatography (HPLC) purification of individual core histones ( Supplementary Fig. 1b ), different combinations of PTMs on full-length H3.1 were identified by top–down FTICR-MS based on the accurate mass measurements [28] ( Supplementary Fig. 1c ). We also used Velos LTQ orbitrap to perform top–down MS ( Supplementary Fig. 2a ) and select ion monitoring (SIM) ETD MS/MS on each of these peaks to sequence the PTM sites on H3. Specifically from non-stimulated BMDMs, through multi-layer SIM ETD MS/MS ‘purification’ ( Supplementary Figs 2b and 3a ) we identified the predominate species in Peak #2 as a multiply modified form of H3.1 containing H3K4me2, K9me2 and K27me2 ( Supplementary Fig. 3b ). Also, an adjacent peak (Peak #1) at 14 Da upfield of Peak #2 contains a mixture with a population carrying an acetylation at lysine 9 (K9ac) along with H3K4me2 and K27me2 (the top panel, Supplementary Fig. 3b ). Notably, the relative K9ac abundance was increased under NL but decreased in TL BMDMs, whereas the opposite in K9me2 abundance was found ( Supplementary Figs 1c and 2a ). Nevertheless, all data identified the key PTM conversion at H3K9 with the TL-specific increase of K9me2 on H3. Because the methylation activity of G9a directly correlates with the accumulation of H3K9me2, combined MS results indicated that, specifically in LPS-tolerized macrophages, G9a promotes acetylation-to-methylation conversion at H3K9. G9a is activated within T-gene chromatins during ET The inflammation-phenotypic PTM change at H3K9 also implied that the H3K9-targeting activity of G9a could be differentially regulated at T-gene promoters in TL versus NL cells. To clarify this, we first performed chromatin immunoprecipitation (ChIP) experiments with anti-K9me2 antibody on the BMDM set under different inflammatory states ( Supplementary Fig. 4a ). Coincident with the MS data ( Supplementary Figs 1–3 ), decreasing dimethylation and increasing acetylation of H3K9 were observed at both distal (cc) and proximal (dd) promoter regions of a T-gene ( IL6 ) under NL. However, in ET macrophages, an increased H3K9me2 was observed at the same regions beyond TSS, indicating that the accumulation/occupancy of H3K9me2 on T-gene promoters during ET introduces a block for both transcription initiation and elongation of T-class genes ( Supplementary Fig. 4b ). Similarly, in ChIP analysis with anti-G9a antibody, dramatically enhanced binding of G9a to the promoter region ‘cc’ and the first intron ‘ee’ was observed during ET ( Supplementary Fig. 4c ), indicating that G9a is recruited to the cis -regulatory elements of IL6 and represses its expression ( Supplementary Fig. 4d ). To clarify the role of G9a in ET-specific dimethylation of H3K9, before LPS stimulation we treated BMDMs with UNC0638 that inhibits the methylation activity of the enzyme but causes little change in its abundance [26] . In ChIP analysis with anti-H3K9me2 antibody, greater decreases in H3K9me2 at the ‘cc’ and ‘ee’ region were observed in the inhibitor pretreated TL cells compared with those under NL ( Supplementary Fig. 4e ). Similar results were obtained from Raw264.7 cells with G9a knockdown ( Supplementary Fig. 4f ); thus upregulation of the methylation activity of G9a correlates with the gene-specific increase in H3K9me2. ChaC enriches active G9a and its phenotypic associators Our ChaC design is based on the fact that UNC0638 specifically binds to the enzymatically active form of G9a (ref. 26 ), aiming to profile the inflammation-phenotypic G9a-interacting proteins within chromatin of differently inflamed macrophages. Meanwhile, the incorporation of amino acid-coded mass tagging (AACT) as in-spectra markers in MS-based quantitative analysis [29] , [30] distinguished protein constituents in the G9a complexes pulled down by UNC0638 from primary BMDMs under different inflammatory states. First we synthesized a UNC0638 derivative, UNC2249, with an aminopropyl linker for coupling UNC0638 to Sepharose beads that retained the same high affinity to G9a as UNC0638 ( Supplementary Fig. 5 and Supplementary Methods ). As illustrated by Fig. 1a , we incubated the UNC0638 beads with nuclear extract from equal amounts of BMDMs under either N ( 13 C-Arg/Lys-labelled, medium) or NL ( 13 C 15 N-Arg/Lys, heavy), or TL (unlabelled, light). While the level of G9a showed a slight decrease in TL cells compared with that in NL macrophages, significantly more G9a was pulled down by UNC2249 from TL cells than from equal amounts of NL cells, indicating higher amounts of chronic-active G9a within the silenced chromatin under ET ( Fig. 1b ). The pull-down proteins from each inflammatory state were mixed in equal proportion based on total protein mass and subjected to nanoLC-MS/MS analysis. In two biological replicates, 2,021 proteins were quantified under NL or TL compared with their abundances in N cells; the ratios of NL/N and TL/N, respectively, represent the relative binding strengths of the corresponding proteins to G9a in either NL or TL compared with binding strength in non-stimulated cells ( Supplementary Data 1 ). Thus, G9a was found to interact with different proteins, or the same proteins with different binding strengths, based on the inflammation-phenotypic methylation activity of G9a in differentially inflamed macrophages ( Fig. 1c ). 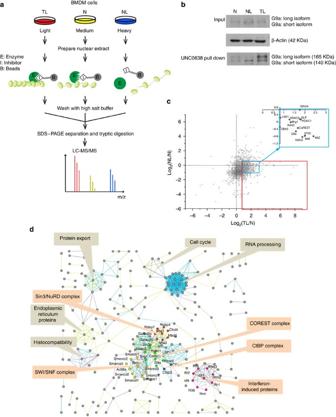Figure 1: Quantitative ChaC for systems dissection of the functional G9a interactome or complexome formed within the chromatin of differentially inflamed macrophages. (a) Workflow of the activity-based ChaC with immobilized UNC0638 coupled with AACT/SILAC quantitative proteomics. Equal amounts of nuclear extract from each set of BMDMs were incubated with Sepharose conjugated with UNC0638 or UNC2249 and the pull-down products were mixed and subjected to LC-MS/MS. (b) Immunoblot analysis of the G9a pulled down by UNC2249 from the BMDMs under different inflammatory conditions (N, NL and TL). Upper bands indicate the long isoform of G9a, while the lower bands are the shorter forms. β-Actin is the loading control. Same in figures below: all full blots are inSupplementary Fig. 14. (c) Scatter plot of the pull-down proteins with TL/N and NL/N ratio measured by AACT-based quantitative ChaC. The insets indicate previously known G9a interactors with their ratios to determine the threshold of NL- or TL-specific interactors. (d) Protein–protein interaction network of TL-specific G9a-interacting protein complexes, determined by STRING in high confidence (The confidence score is at 0.7). Figure 1: Quantitative ChaC for systems dissection of the functional G9a interactome or complexome formed within the chromatin of differentially inflamed macrophages. ( a ) Workflow of the activity-based ChaC with immobilized UNC0638 coupled with AACT/SILAC quantitative proteomics. Equal amounts of nuclear extract from each set of BMDMs were incubated with Sepharose conjugated with UNC0638 or UNC2249 and the pull-down products were mixed and subjected to LC-MS/MS. ( b ) Immunoblot analysis of the G9a pulled down by UNC2249 from the BMDMs under different inflammatory conditions (N, NL and TL). Upper bands indicate the long isoform of G9a, while the lower bands are the shorter forms. β-Actin is the loading control. Same in figures below: all full blots are in Supplementary Fig. 14 . ( c ) Scatter plot of the pull-down proteins with TL/N and NL/N ratio measured by AACT-based quantitative ChaC. The insets indicate previously known G9a interactors with their ratios to determine the threshold of NL- or TL-specific interactors. ( d ) Protein–protein interaction network of TL-specific G9a-interacting protein complexes, determined by STRING in high confidence (The confidence score is at 0.7). Full size image We then investigated the quantitative threshold that distinguishes ET-specific G9a-associating proteins. First, log 2 (TL/N) or log 2 (NL/N) of G9a was found at 1.58 or −0.52, respectively, which was a similar trend with the inflammation-phenotypic changes in the methylation activity of G9a ( Supplementary Fig. 4e,f ). Second, based on the ratios for multiple proteins known to co-exist with G9a in various complexes, such as HP1 (ref. 10 ), GLP, histone deacetylase (HDAC1), HDAC2, LSD1/KDM1A, WIZ, SIN3A and Brg1, the threshold to distinguish TL-specific G9a interactors was empirically determined as the borderline ratios with log 2 (TL/N)>0.82 and log 2 (NL/N)<0.68 or log 2 (TL/NL)>1 ( Fig. 1c and Supplementary Figs 6 and 7 ), that is, the associations between G9a and these proteins are enhanced specifically in TL cells but weakened or non-specific under NL. Notably, in contrast to the relatively poor-correlated ratios of NL/N for the proteins quantified by biological replicates, the TL/N ratios of these proteins showed good reproducibility with correlation of linearity ( R value at 0.82; Supplementary Fig. 8a ). To validate the physiological accuracy of ChaC-identified proteins, we examined whether their recruitment onto T-gene promoters is truly dependent on chronic-active G9a. We generated paired Raw264.7 cell lines with either stable short hairpin RNA (shRNA)-mediated G9a knockdown (KD) or its wild-type counterpart Raw264.7 cells transfected with the empty vector (EV; Supplementary Fig. 9a ), from which the results are compared with the UNC0638-treated primary BMDMs under defined inflammatory conditions. First, given that HDAC1 is a shared component of multiple complexes pulled down with G9a specifically during ET, we examined by ChIP–PCR the inflammation-phenotypic binding of HDAC1 to a T-gene ( IL6 ) promoter. Compared with wild-type Raw264.7 cells under NL, IL6 -specific binding of HDAC1 was increased during ET, which was then diminished in either G9a-KD cells or UNC0638-treated BMDMs ( Fig. 2a ). Thus, the ET-specific recruitment of HDAC1 at the T-class promoter is dependent on chronic-active G9a. Conversely, recruitment of G9a was affected by HDAC, as the abundance of G9a was reduced within the T-class promoters in the TL cells pretreated by the HDAC inhibitor SAHA ( Fig. 2b ), implying a coordinated action between both histone-modifying enzymes when HDAC removes the acetyl group at H3K9 to facilitate accessibility of G9a. Meanwhile, SirT-1, a substrate of G9a (ref. 18 ), which plays a deacetylation role during ET [31] , [32] , was also quantified as a TL-specific G9a associator (1.1, −0.88), and showed a similar enrichment on IL6 as HDAC1, indicating both play the redundant role in K9 deacetylation ( Supplementary Fig. 9c ). Previous work showed the LPS-induced recruitment of Brg1, a key component of chromatin remodelling complex, on T-genes was attenuated under TL [7] . However, in the G9a-depleted cells, recruitment of Brg1 was recovered on the IL6 distal promoter region, indicating that G9a plays a crucial role in determining Brg1 occupation within the T-gene chromatin while G9a co-exists with Brg1 in the SWI/SNF complexes ( Fig. 2c ). Notably, the consistent observations in G9a KD Raw264.7 cells versus UNC0638-treated BMDMs demonstrated the high specificity of UNC0638 in binding to the chronic-active G9a that coordinates assembly of a repressome within the silenced, LPS-tolerant chromatin. 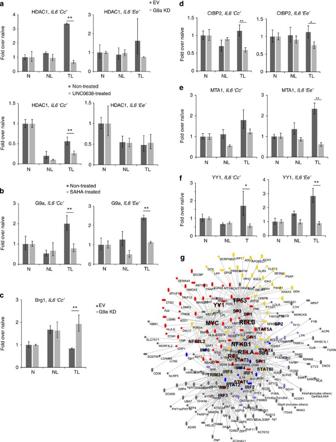Figure 2: Recruitment of TL-specific G9a associates to the chromatin of T-class gene promoters is G9a dependent. ChIP assay was performed in (a, upper) paired wild-type versus G9a KD Raw264.7 cells, with the antibody against HDAC1, (a, lower) ChIP assay against HDAC1 in BMDMs with or without UNC0638 treatment. (b) ChIP assay against G9a antibody in BMDMs with or without SAHA treatment. ChIP assay was performed in paired wild-type versus G9a KD Raw264.7 cells, with the antibody against Brg1 (c), CtBP2 (d), MTA1 (e), YY1 (f) to measure their binding toIL6proximal promoter (‘Cc’) and intragenic (‘Ee’) regions. EV served as the control line. Same in figures below: error bars that represent the mean of triplicates were obtained as follows: an upper error bar was determined by 2−(dCt−SD)−2−(dCt), and the lower one was by 2−(dCt)−2−(dCt+SD). *P<0.05 gives the statistical significant difference of ChIP–PCR enriched gene between two defined cell conditions according to two-tailed unpaired Student’st-test. **P<0.01 (g) The co-regulatory network is composed of multiple transcription factors identified by ChaC and their downstream genes identified by G9a-dependent quantitative proteomics. Rectangles represent transcription factors and filled circles represent targeting genes. Figure 2: Recruitment of TL-specific G9a associates to the chromatin of T-class gene promoters is G9a dependent. ChIP assay was performed in ( a , upper) paired wild-type versus G9a KD Raw264.7 cells, with the antibody against HDAC1, ( a , lower) ChIP assay against HDAC1 in BMDMs with or without UNC0638 treatment. ( b ) ChIP assay against G9a antibody in BMDMs with or without SAHA treatment. ChIP assay was performed in paired wild-type versus G9a KD Raw264.7 cells, with the antibody against Brg1 ( c ), CtBP2 ( d ), MTA1 ( e ), YY1 ( f ) to measure their binding to IL6 proximal promoter (‘Cc’) and intragenic (‘Ee’) regions. EV served as the control line. Same in figures below: error bars that represent the mean of triplicates were obtained as follows: an upper error bar was determined by 2 −( dCt −SD) −2 −( dCt ) , and the lower one was by 2 −( dCt ) −2 −( dCt+ SD) . * P <0.05 gives the statistical significant difference of ChIP–PCR enriched gene between two defined cell conditions according to two-tailed unpaired Student’s t -test. ** P <0.01 ( g ) The co-regulatory network is composed of multiple transcription factors identified by ChaC and their downstream genes identified by G9a-dependent quantitative proteomics. Rectangles represent transcription factors and filled circles represent targeting genes. Full size image Chronic-active G9a is at the core of a repressome complex Meeting the quantitative criteria above, 606 proteins were identified as TL-specific G9a interactors, which are predominantly clustered in functions such as DNA methylation, mRNA processing, transcriptional repression and macromolecule metabolism ( Supplementary Fig. 8c ). Further, by using STRING to explore the protein–protein interaction network, among these TL-specific G9a-interacting proteins, a few functional clusters that contain the intensive interactions were identified, indicating these canonical pathways/programs are interactive during ET ( Fig. 1d ). We also identified multiple factors previously known as components of CoREST complex [13] , CtBP complex [14] , SWI/SNF chromatin remodelling complexes [15] and NuRD complex [16] . For example, HDAC2, LSD1, Brg1, SIN3A and G9a ( Fig. 1c ) are the known components of CoREST complex, a transcriptional repressor module [13] . Simultaneously, a few proteins associated with carbohydrate metabolic processes, such as GRP78 and UGGG1, were identified, consistent with that CtBP is a NADH-dependent transcriptional repressor that links carbohydrate metabolism to epigenetic regulation by recruiting diverse histone-modifying complexes [33] . Further, we identified WIZ, a known substrate of G9a, which links the G9a/GLP heteromeric complex to the CtBP co-repressor machinery [34] . Accordingly ChIP–PCR validated that recruitment of CtBP2 within the T-class promoter was G9a dependent during ET ( Fig. 2d ). In the same pull-down complexome ( Supplementary Data 1 ), multiple components/subunits of ATP-dependent chromatin remodelling complexes and NuRD, were found to interact with chronic-active G9a. Given that the G9a-mediated methylation of MTA1, a key component of NuRD, is required for repression by NuRD [35] , we also employed ChIP–PCR to investigate the G9a-dependent recruitment of the NuRD complex during ET and observed that the enhanced TL-specific binding of MTA1 to T-class genes was diminished in either G9a-KD Raw cells or UNC0638-treated BMDMs ( Fig. 2e ), indicating the chronic-active G9a determines the stability of a functional NuRD repressor complex within T-chromatin. To partly explore the functional implication of the TL-specific G9a interactions, we compared the data set of UNC2249/UNC0638 pull-down proteins from TL BMDMs with the documented list of G9a non-histone substrates. Eight out of 16 proteins, including ACINUS, C/EBPt and WIZ that were the known G9a substrates, were found in the UNC2249 pull-down complex ( Supplementary Table 1 ). Further, the TL-specific interactome constructed based on the UNC2249 pull-down data showed significant overlap with what was mapped based on the G9a-target Kme proteome [18] , [36] ( Supplementary Fig. 8d ), indicating that these proteins are the inflammation-phenotypic substrates of chronic-active G9a. Notably, although UNC0638 is a G9a substrate-competitive inhibitor, certain G9a substrates were pulled down probably due to their roles as the co-factors associating with other proteins that directly interact with the enzymatically active G9a, implicating that chronic-active G9a broadly facilitates the TL-specific complex assembly by modulating Kme-dependent protein–protein interactions. Meanwhile, many proteins previously unknown to associate with G9a were identified during ET, generating multiple hypotheses that extend current knowledge of the mechanisms involved in the transcriptional regulation of ET. Chronic-active G9a interacts with select HMTases during ET For the first time, ChaC revealed an enhanced association between the H3K36-targeting HMTase NSD3 and G9a specifically in ET cells ( Fig. 1c ), which was validated by an in vitro co-immunoprecipitation experiment ( Fig. 3a ), implicating the cooperative action of both HMTases during ET. Further, to clarify whether the H3K36-targeting methylation activity of NSD3 depends on chronic-active G9a, we compared the abundance of dimethylated H3K36 in either paired wild-type versus G9a-KD Raw264.7 macrophages or non-treated versus UNC0638-treated BMDMs. Compared with its TL-specific increase in wild-type cells, the level of H3K36me2 decreased in either G9a-KD or UNC0638-treated cells ( Fig. 3b ), indicating that both the methylation activity of NSD3 and the deposition of the K36me2 code on H3 are G9a-dependent during ET. Notably, the methylated level of H3K27 was also reduced in G9a-KD or UNC0638-treated cells in line with a report that G9a also targets H3K27 (ref. 37 ). In addition, the TL-specific enrichment of NSD3 at the IL6 promoter was found dependent on chronic-active G9a ( Fig. 3c ), revealing that chronic-active G9a also coordinates the combinatorial deposition of multiple Kme codes on H3 by recruiting NSD3 into T-chromatin. Further, a recent report indicated that both NSD3 and G9a participate in LSD2 complex for regulating transcription elongation by modulating intragenic H3K4me2 [38] , supporting our findings of the co-existence of both G9a and NSD3 in the TL-specific complexome. Meanwhile, ASH2l, another HMTase that catalyses H3K4 trimethylation for transcriptional activation and is also a core member of the transcription-initiating COMPASS/COMPASS-like complexes [39] , was identified along with other members of COMPASS, WDR82 and CXXC1 ( Supplementary Table 2 ). The enhanced interaction between G9a and ASH2l in ET macrophages was also validated by co-transfection and co-IP experiments ( Fig. 3d ). Further, even in the LPS-tolerant macrophages, G9a showed a higher affinity to the peptide containing H3K4me2 than to its unmodified counterpart, while the H3K4me2/3 level was little changed across all inflammatory conditions ( Fig. 3e ). Thus, following acute stimulation, G9a may become chronically active by first docking on ASH2l-target H3K4me3 deposited in the transcriptional-active chromatin associated with T-genes. 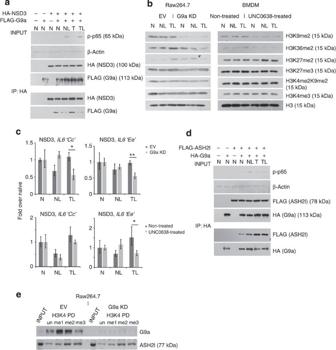Figure 3: Chronic-active G9a interacts with select HMTases during ET. NSD3 (a) and ASH2L (d) specifically interact with chronically active G9a in LPS-tolerant 293-TLR4/CD14/MD2 cells. Cell responses were monitored by p65 phosphorylation. (b) Lysine methylation at multiple sites on H3 was compared in paired wild-type or G9a KD Raw264.7 cells (left) and in BMDMs with or without 2-day UNC0638 treatment (right). Unmodified H3 was used as the loading control. (c) ChIP assay of NSD3 deposition onIL6‘Cc’ and ‘Ee’ region in the same sample pairs as (b). *P<0.05; **P<0.01. Two-tailed unpaired Student’st-test. (e) Immunoblot analysis of the pulled down products from a paired wild-type versus G9a KD Raw264.7 cells under TL using histone H3 lysine 4 methylated peptides. Figure 3: Chronic-active G9a interacts with select HMTases during ET. NSD3 ( a ) and ASH2L ( d ) specifically interact with chronically active G9a in LPS-tolerant 293-TLR4/CD14/MD2 cells. Cell responses were monitored by p65 phosphorylation. ( b ) Lysine methylation at multiple sites on H3 was compared in paired wild-type or G9a KD Raw264.7 cells (left) and in BMDMs with or without 2-day UNC0638 treatment (right). Unmodified H3 was used as the loading control. ( c ) ChIP assay of NSD3 deposition on IL6 ‘Cc’ and ‘Ee’ region in the same sample pairs as ( b ). * P <0.05; ** P <0.01. Two-tailed unpaired Student’s t -test. ( e ) Immunoblot analysis of the pulled down products from a paired wild-type versus G9a KD Raw264.7 cells under TL using histone H3 lysine 4 methylated peptides. Full size image Chronic-active G9a promotes gene-specific co-repression From the silenced chromatin of LPS-tolerized BMDMs, we also found that UNC2249/UNC0638 selectively enriched/pulled down a cluster of low-abundance transcriptional factors (TFs) or DNA-binding proteins ( Supplementary Table 3 ). 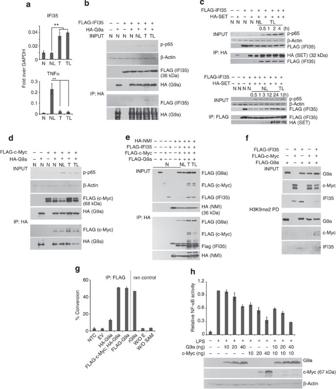Figure 4: Chronically active G9a forms a stable complex with IFI35, NMI, and c-Myc during ET. (a) IFI35 remained active in LPS-tolerant cells. mRNA expression was normalized to GAPDH. The release of TNFα indicates the strength of immune response. **P<0.01. Two-tailed unpaired Student’st-test. (b) and c-Myc (d) specifically interact with G9a in LPS-tolerant, TLR4/CD14/MD2 293 cells. (c) IFI35 interacts with the catalytic SET domain of G9a in TL cells as assayed by IP with HA-tagged SET (upper), and vice versa (lower). (e) NMI, IFI35, c-Myc and G9a were co-immunoprecipitated from LPS-tolerant cells. (f) Both IFI35 and c-Myc associate with the peptide containing H3K9me2 in the complex with G9a. (g) c-Myc promotes the HMTase activity of G9a. c-Myc and G9a were co-transfected into LPS-tolerant, TLR4/CD14/MD2 293 cells and c-Myc was enriched for the H3K9 HMTase activity assay. ‘NTC’ refers to non-transfected control cells, EV is the EV control, HA-G9a represents the IP background and FLAG-G9a is a positive control for HMTase activity. Recombinant G9a (rG9a) is a positive control forin vitroreactions, and the reactions either without enzyme (W/O E) or without S-adenosyl methionine (W/O SAM) are negative controls. (h) G9a significantly repressed NF-κB reporter genes in a dose-dependent manner in cooperation with c-Myc. All luciferase assays were performed with three individual preparations. Values and error bars indicate the mean and s.d. among biological triplicates. The ectopic proteins were detected by immunoblotting. β-Actin is the loading control. Notably, both transcriptional repressive subunits of the NF-κB family, RelB and C-Rel were identified specifically in the chronic-active G9a complexome, while other NF-κB subunits including p65 and p100/p105 were identified with random, lower TL/N ( Supplementary Table 4 ). Meanwhile, ChIP experiments showed NL-specific recruitment of p65 to T-genes ( Supplementary Fig. 10 ), indicating the dissociation of the inflammation-activating NF-κB subunit(s) from the silenced T-gene chromatin, while repressive NF-κB was selectively recruited into the TL-specific complexome. In addition, a transcriptional repressor YinYang1(YY1) that was implicated in mediating transcriptional repression by interacting with either CtBP [40] , Sin3 or HDACs [41] , was also identified as a TL-specific complexome component. Recent work [42] indicated that NF-κB-dependent increased YY1 expression negatively regulates interferon (IFNβ) production, possibly mediated by C-Rel and RelB. Importantly, here, YY1 was found together with these co-repressor complex components or transcriptional repressors during ET. Accordingly, the existence of YY1 at T-gene ( IL6 ) promoters was found dependent on G9a in ET macrophages ( Fig. 2f ), indicating that chronic-activated G9a facilitates the simultaneous access of select TFs to T-gene promoters during ET. To determine the impact of the co-recruitment of combinatorial TFs with G9a on gene-specific expression during ET, we conducted AACT-based quantitative proteomics [29] , [30] on paired wild-type and G9a-KD Raw264.7 macrophages under TL to identify/profile the global, differential proteome expression caused by G9a depletion. In LPS-tolerant macrophages, 421 out of 5,393 quantifiable proteins showed G9a-repressed expression by more than 2-fold; statistically over-represented in gene ontology function clusters for immune response, apoptosis and cell proliferation ( Supplementary Fig. 9b ). By using Ingenuity Pathway Analysis, we identified a well-connected gene regulatory network among 198 G9a-repressing proteins that were previously known gene products regulated by either one or several of select TFs ( Fig. 2g ). Importantly, many of these proteins at the network nodes are regulated by multiple TFs, indicating that these TFs that are selectively recruited with chronic-active G9a work in concert to co-regulate their target genes. These data reveal that chronic-active G9a extends its repressive role in the chromatin-associated, gene-specific regulation of ET by coordinating the co-regulatory action of select transcriptional repressors. Chronic-active G9a interacts with IFN-inducible complexes Strikingly, a cluster of IFN-inducible proteins including IFN-inducible protein 35 (IFI35) and N-myc-interactor (Nmi) was identified as TL-specific, G9a-interacting proteins ( Fig. 1c ). Both the involvement of G9a in IFN signalling [43] and H3K9me2 as an epigenetic signature of IFN/cytokine signalling [44] were suggested. Therefore, we reasoned that chronic-active G9a interacts with this cluster of proteins to extend its function in under-characterized regulatory pathway(s) for gene-specific regulation during ET. Except for its role in the transcription repression mediated by c-Myc oncogene [45] , the function of IFI35 in inflammation control is ambiguous. First we found that the expression of IFI35 remained LPS-inducible even under ET ( Fig. 4a ), showing the typical feature of non-tolerizable (NT)-class genes [6] . Meanwhile, G9a-IFI35 association was significantly enhanced during ET ( Fig. 4b ). Further, the catalytic SET domain of G9a was found directly involved in the ET-specific G9a-IFI35 interaction ( Fig. 4c ), suggesting a determining role of G9a methylation activity in coordinating the IFN-inducible complex specifically during ET. Figure 4: Chronically active G9a forms a stable complex with IFI35, NMI, and c-Myc during ET. ( a ) IFI35 remained active in LPS-tolerant cells. mRNA expression was normalized to GAPDH. The release of TNFα indicates the strength of immune response. ** P <0.01. Two-tailed unpaired Student’s t -test. ( b ) and c-Myc ( d ) specifically interact with G9a in LPS-tolerant, TLR4/CD14/MD2 293 cells. ( c ) IFI35 interacts with the catalytic SET domain of G9a in TL cells as assayed by IP with HA-tagged SET (upper), and vice versa (lower). ( e ) NMI, IFI35, c-Myc and G9a were co-immunoprecipitated from LPS-tolerant cells. ( f ) Both IFI35 and c-Myc associate with the peptide containing H3K9me2 in the complex with G9a. ( g ) c-Myc promotes the HMTase activity of G9a. c-Myc and G9a were co-transfected into LPS-tolerant, TLR4/CD14/MD2 293 cells and c-Myc was enriched for the H3K9 HMTase activity assay. ‘NTC’ refers to non-transfected control cells, EV is the EV control, HA-G9a represents the IP background and FLAG-G9a is a positive control for HMTase activity. Recombinant G9a (rG9a) is a positive control for in vitro reactions, and the reactions either without enzyme (W/O E) or without S-adenosyl methionine (W/O SAM) are negative controls. ( h ) G9a significantly repressed NF-κB reporter genes in a dose-dependent manner in cooperation with c-Myc. All luciferase assays were performed with three individual preparations. Values and error bars indicate the mean and s.d. among biological triplicates. The ectopic proteins were detected by immunoblotting. β-Actin is the loading control. Full size image Except for c-Myc, other proteins in the complexes of STATs and Myc proteins [46] were all identified as TL-specific G9a-interacting partners. To test the conjecture that failure to detect c-Myc was due to its high-turnover rate, we examined the in vitro , inflammation-phenotypic interaction of G9a with c-Myc as well as with other proteins. Consistent with TL-specific G9a-c-Myc interaction ( Fig. 4d ), all four proteins enhanced their association in the same complex immunoprecipitated from the LPS-tolerant cells co-transfected with four epitope-tagged constructs respectively expressing IFI35, G9a, c-Myc, Nmi ( Fig. 4e ). Further, these associations were promoted by both G9a and H3K9me2, as the complex involving all components was pulled down only from the co-transfected cells under TL using a H3K9me2-containing peptide ( Fig. 4f ). Thus, both chronic-active G9a and H3K9me2 are required for the integrity of IFI35/c-Myc/Nmi complex that specifically recognizes/docks on H3K9me2 during ET. We further investigated whether c-Myc impacts the function of G9a during ET by measuring the methylation activity of G9a with or without over-expressing c-Myc. We transfected epitope-tagged G9a or co-transfected both c-Myc and G9a into the stable TLR4-expressing cells under TL. With a H3 amino-terminal peptide as the substrate, HMTase activity increased with the co-expression of both proteins, indicating that c-Myc is a part of the complex involving chronic-active G9a ( Fig. 4g ). We then investigated the impact of this G9a/K9me2-dependent complex on NF-κB-dependent transcription. An NF-κB-target luciferase reporter was co-transfected with the expression vector(s) of either G9a, or c-Myc, or both. As shown in Fig. 4h , LPS-induced NF-κB activity decreased with increasing expression of either G9a or c-Myc, while IFI35 and Nmi had little effect on G9a/c-Myc-associated suppression of NF-κB activity ( Supplementary Fig. 11 ), indicating that c-Myc and chronic-active G9a work synergistically to suppress pro-inflammatory NF-κB activity during ET. Also, this G9a-dependent suppression of NF-κB activity is readily interpreted by our observation of the G9a-dependent existence of RelB, the repressive subunit of NF-κB, in the T-gene nucleosome during ET ( Supplementary Table 4 ). c-Myc regulates G9a-dependent gene-specific transcription Myc broadly targets more than 1,500 genes involving in diverse biological processes [47] . To uncover G9a-dependent, c-Myc-regulated pathways/processes, we performed ChIP-seq experiments using anti-c-Myc antibody on paired wild-type and G9a-KD Raw264.7 cells under TL. Comparative genome-wide mapping of c-Myc binding loci was obtained to identify the G9a-dependent occupancy of select c-Myc-regulated genes ( Fig. 5a ). G9a knockdown led to decreased binding of c-Myc to 1,132 genes, including a number of T-genes such as IL10 , Lipg , Itga4 and apoptosis-related genes including Bax and Bcl2l2-Pabpn1 ( Fig. 5b ). For instance, the enrichment of c-Myc at the IL10 distal promoter was found in wild-type but not in G9a-KD cells. No peak was found in the proximal promoter of IL10 in either wild-type or G9a-KD cells, consistent with the results from ChIP–PCR validation ( Fig. 5c ). Notably, 38% of the G9a-depedent, c-Myc binding genes identified by ChIP-seq are c-Myc-regulated genes found in fibroblasts and B-lymphoid tumour cells [48] , [49] ( Supplementary Data 2 ), indicating that c-Myc also contributes to ET through regulating select genes in the G9a-dependent manner. Further, ChIP-qPCR validated the dual dependence of other known T-class or NT-class genes. For example, c-Myc showed enhanced binding to the loci of IL6 specifically under TL, which was diminished consistently in either UNC0638-treated BMDMs or G9a-KD Raw264.7 cells ( Fig. 5d ). c-Myc binding to the NT genes was not affected by either the inhibitor or G9a-KD, all demonstrating that the TL-specific recruitment/accessibility of c-Myc to T-gene promoters is dependent on chronic-active G9a. As well, along with additional recruitment of c-Myc to IL6 , IP-10 , and p21 (the universal cell cycle inhibitor p21 cip ) (ref. 50 ) in the wild-type cells under TL compared with NL, short interfering RNA-mediated knockdown of G9a or UNC0638 inhibition of chronic-active G9a led to reduced c-Myc binding to these genes. Given the pro-inflammatory nature of IL6 , this result suggested that the G9a-dependent binding of c-Myc to T-gene promoters is responsible for the suppression of this class of the genes during ET. Further, given that both IP-10 and p21 are known c-Myc-regulated genes involved in cell survival, we concluded that chronic-active G9a extends its epigenetic repressive role in cell fate decision by regulating the transactivation activity of c-Myc during the inflammation control of ET. 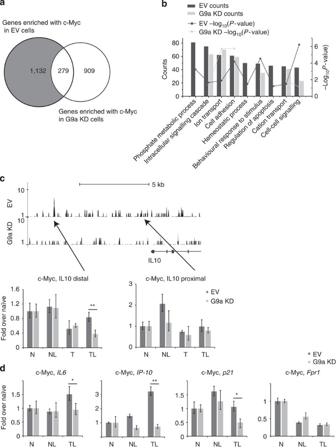Figure 5: Genomic mapping of G9a-dependent c-Myc binding targets. (a) Schematic Venn diagram represents the overlap of c-Myc binding genes between G9a KD and the wild-type (EV) cells. c-Myc binding peaks located between 10 kb upstream from the start site and 10 kb downstream from the stop site of annotated transcripts are considered as gene-relevant bindings. (b) Gene ontology biological process analysis indicates the clusters over-represented in the c-Myc binding genes from G9a KD and wild-type cells, respectively. (c) Representative images depict c-Myc ChIP-seq binding profiles onIL10genome (upper). c-Myc deposition was validated by ChIP assay onIL10distal and proximal promoter regions in G9a KD and wild-type cells (lower). (d) ChIP assay of c-Myc binding onIL6,IP-10, p21andFpr1promoters in G9a KD and wild-type cells. *P<0.05; **P<0.01. Two-tailed unpaired Student’st-test. Figure 5: Genomic mapping of G9a-dependent c-Myc binding targets. ( a ) Schematic Venn diagram represents the overlap of c-Myc binding genes between G9a KD and the wild-type (EV) cells. c-Myc binding peaks located between 10 kb upstream from the start site and 10 kb downstream from the stop site of annotated transcripts are considered as gene-relevant bindings. ( b ) Gene ontology biological process analysis indicates the clusters over-represented in the c-Myc binding genes from G9a KD and wild-type cells, respectively. ( c ) Representative images depict c-Myc ChIP-seq binding profiles on IL10 genome (upper). c-Myc deposition was validated by ChIP assay on IL10 distal and proximal promoter regions in G9a KD and wild-type cells (lower). ( d ) ChIP assay of c-Myc binding on IL6 , IP-10, p21 and Fpr1 promoters in G9a KD and wild-type cells. * P <0.05; ** P <0.01. Two-tailed unpaired Student’s t -test. Full size image Chronic-active G9a inhibits c-Myc degradation during ET Given our newly characterized, broad effect of c-Myc on transcriptional co-regulation, we next investigated how chronic-active G9a regulates c-Myc during ET. We first compared the inflammation-phenotypic expression of c-Myc in wild-type versus G9a-KD Raw264.7 cells ( Fig. 6a ). For wild-type cells, compared with its abundance under N or NL, slightly less c-Myc was observed under TL. Although little change was found for both wild-type and G9a-KD cells under N or NL, the abundance of c-Myc was substantially lower in the TL G9a-KD cells, suggesting the role of chronic-active G9a in maintaining the abundance of c-Myc in LPS-tolerant macrophages. We then determined at what levels G9a regulates c-Myc stability. First, RT-PCR showed that c-Myc mRNA was elevated in G9a-depleted cells, suggesting that G9a suppresses c-Myc transcription ( Fig. 6b ). Second, the rate of c-Myc decay following inhibition of protein synthesis with cycloheximide was about four times slower in the TL wild-type cells than in the G9a KD counterpart ( Fig. 6c ). Also, more c-Myc was detected with increasing expression of G9a ( Supplementary Fig. 12a,b ), indicating that chronic-active G9a stabilizes c-Myc at T-gene promoters by inhibiting c-Myc degradation during ET. Further, we pretreated either wild-type or G9a-KD cells with the proteasome inhibitor MG-132, which allowed analysis of the time-dependent translation of c-Myc mRNA when protein degradation was blocked. In contrast to the time-dependent, progressive accumulation of c-Myc in G9a-KD cells, the MG-132-induced c-Myc was actually reduced with a longer post-treatment time in the presence of G9a ( Fig. 6d ), indicating that G9a also attenuates c-Myc translation, consistent with the TL-specific decrease of c-Myc in the wild-type cells ( Fig. 6a ). Thus, G9a-dependent inhibition of c-Myc degradation at the post-translational level is the predominate process that determines the stability and then the accessibility of c-Myc onto T-gene promoters. 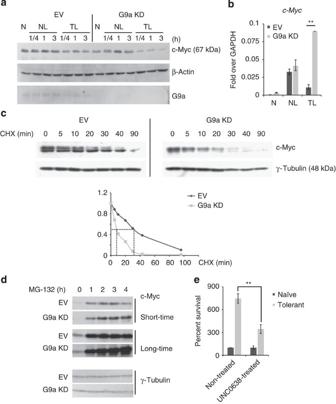Figure 6: Chronically active G9a stabilizes c-Myc and promotes cell survival. (a) c-Myc protein expression was diminished in G9a KD cells under TL conditions. The abundance of G9a was measured to determine G9a knockdown efficiency and β-Actin was the loading control. (b) c-Myc mRNA expression was elevated in G9a KD, LPS-tolerant cells, represented by the relative expression normalized to GAPDH. (c) c-Myc half-life was measured in wild-type (EV) and G9a KD tolerant cells treated with cycloheximide (CHX) in a time-dependent manner. The intensities of c-Myc are shown asyvalue in the scatter plot, and c-Myc half-life was indicated by crossing dashed line withxaxis. γ-Tubulin is the loading control. (d) c-Myc accumulation was investigated by applying a time-course MG-132 treatment on LPS-tolerant cells. (e) Activated G9a is required to maintain cell survival in tolerant cells. Cell viability was measured as survival percentage normalized to non-treated naïve cells. **P<0.01. Two-tailed unpaired Student’st-test. Figure 6: Chronically active G9a stabilizes c-Myc and promotes cell survival. ( a ) c-Myc protein expression was diminished in G9a KD cells under TL conditions. The abundance of G9a was measured to determine G9a knockdown efficiency and β-Actin was the loading control. ( b ) c-Myc mRNA expression was elevated in G9a KD, LPS-tolerant cells, represented by the relative expression normalized to GAPDH. ( c ) c-Myc half-life was measured in wild-type (EV) and G9a KD tolerant cells treated with cycloheximide (CHX) in a time-dependent manner. The intensities of c-Myc are shown as y value in the scatter plot, and c-Myc half-life was indicated by crossing dashed line with x axis. γ-Tubulin is the loading control. ( d ) c-Myc accumulation was investigated by applying a time-course MG-132 treatment on LPS-tolerant cells. ( e ) Activated G9a is required to maintain cell survival in tolerant cells. Cell viability was measured as survival percentage normalized to non-treated naïve cells. ** P <0.01. Two-tailed unpaired Student’s t -test. Full size image G9a suppresses cell response and gene-specific secretion To further clarify the impact of G9a-mediated stabilization of c-Myc on cell fate decision during ET, we pretreated wild-type and G9a-KD cells with UNC0638 and chronically stimulated them with LPS. While little effect of UNC0638 treatment was observed for the non-treated wild-type cells, the relatively high percentage of survived cells under TL was reduced in cells pretreated with UNC0638 ( Fig. 6e ). Thus, UNC0638 could resensitize ET macrophages and promote their apoptosis by inhibiting chronic-active G9a, revealing that c-Myc plays a cooperative role with TL-specific G9a complexome, the IFN signalling cluster in particular, in regulating ET. We further investigated the impact of chronic-active G9a on gene-specific transcription and translation. First, we employed a label-free quantitative proteomic method for profiling BMDM secretome [51] to identify the proteins differentially secreted from the BMDMs under N, NL, TL without or with UNC0638 treatment, respectively. As a result, the secretion levels of 45% of a total of 992 identified proteins showing repressed releases was found increasing in the UNC0638-pretreated BMDMs under TL ( Supplementary Fig. 13a ). RT-PCR analysis of some of these T-genes or 18 out of 31 selected genes also showed the similar trend of G9a-dependent changes ( Supplementary Fig. 13b ), all indicating that chronic-active G9a broadly affects on the endotoxin-induced transcription and translation of select pro-inflammatory/T-class genes. Because protein complexes are immunoprecipitated based on the abundance and not the activity of the bait protein [19] , conventional antibody-dependent approaches for interactome screening are less sensitive/accurate in distinguishing in situ functional interactions. Here we present a breakthrough in introducing an activity-based ChaC methodology to reveal the inflammation-phenotypic, functional constituents of the chromatin writer complexome that regulates the gene-specific transcription. Unlike most ABPP inhibitors that bind to the active site of their target enzymes, our ChaC chemoprobe is a substrate-competitive ligand, so that the G9a-scaffolding function to accommodate the functionally relevant protein interactions is preserved. Further, because of its high specificity in binding to active G9a, both antibody specificity and cross-activity are no longer the concerns. First, our characterization of HDAC1, SirT-1 and Brg1 as the TL-specific G9a-associating partners ( Fig. 2c ) support the idea that chronic-active G9a holds up particular chromatin remodelling complexes within the silenced chromatin, and, in parallel, both HDAC1 (ref. 14 ) and SirT-1 are recruited to chromatin and then works in concert with chronic-active G9a to promote the phenotypic PTM conversion at H3K9 ( Supplementary Figs 1c and 2a ). Second, in the TL-specific complexome, G9a interacts with select writer(s) or eraser(s) of these methyl-lysine sites, leading to concerted changes of multiple methyl-lysine marks ( Fig. 3 ). The constitutive interaction between ASH2l and G9a ( Fig. 3d ) provided an interpretation for the previous finding that G9a targets H3K9 at the euchromatic regions demarcated by K4me2/3 where G9a is first recruited to the transcriptional-activated regions to later suppress transcription of T-genes [11] . H3K4me2/3 plays a critical auxiliary role, which is maintained by the G9a-ASH2l interaction. Here our combined results provide a systems view that, during ET, chronic-active G9a coordinates deposition of combinatorial Kme sites on H3 known to play either an individual or combinatorial role in gene suppression [52] to synergistically maintain a repressive chromatin landscape at T-gene promoters. In tumour cells, c-Myc is an oncogenic transcriptional activator [47] that preferentially targets genes enriched with the transcriptional-active codes, such as H3K4me2/3 and H3K9ac, through interaction with a variety of histone acetyltransferase (HAT)-associated protein complexes where c-Myc is also a substrate of defined HATs and can be stabilized by acetylation [53] . Conversely, little is known about how the transcriptional activity of c-Myc is regulated during inflammation control. We are the first to find that, specifically in ET macrophages, c-Myc interacts with G9a in an IFI35/c-Myc/Nmi complex that can dock on the transcriptional repressive mark of H3K9me2. Multiple c-Myc-regulated genes were also identified in the G9a-dependent co-regulatory network involving a combinatorial set of transcriptional repressors, indicating that c-Myc is a major component of the G9a repressome ( Fig. 2g ). Further, given that c-Myc is expressed ubiquitously, and its stability is essential for its transcriptional activity, our finding that chronic-active G9a stabilizes c-Myc within promoters of select genes implicates the G9a-dependent role of c-Myc in transcriptional repression during ET. Therefore, c-Myc is a dual-functional TF, alternatively acting as either an activator or a repressor based on its epigenetic environment involving interacting histone codes and select histone-modifying enzymes. During ET c-Myc becomes a G9a/H3K9me2-dependent transcriptional repressor in a similar way as it acts as a HAT/K9ac-dependent transcriptional activator ( Fig. 7a ). This conclusion is also supported by reports that c-Myc plays a regulatory role in anti-inflammatory macrophages [54] and it interacts with a G9a-associating factor Gfi-1 at the p21-promoter region to epigenetically repress p21 (ref. 55 ), indicating that the epigenetic mechanisms dictate the phenotypic binding of c-Myc to select target genes. Further, the global profiling of G9a-regulated protein expression together with ChIP-seq to identify the regulatory DNA elements reveal select genes showing the dual dependence on both G9a and c-Myc during the ET phenotype. These genes mostly fall into the over-represented functional categories associated with immune or inflammatory response, and apoptosis, demonstrating exactly how G9a coordinates the gene-specific regulation of chronic inflammation through the methylation activity-based complexome assembly. 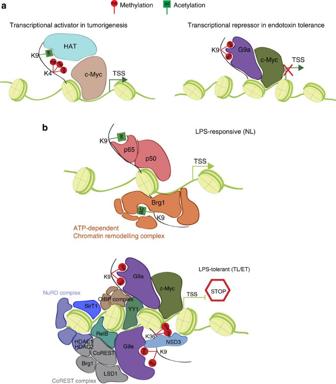Figure 7: The mechanistic models of G9a-dependent, gene-specific regulation of transcription. (a) c-Myc is a dual-functional transcription factor dependent upon either an acetyl-lysine or methyl-lysine-enriched environment when chronically active G9a promotes its transcriptional activity to repress select genes. (b) Chronically active G9a selectively recruits defined protein complexes into the chromatin of pro-inflammatory genes for their silencing during ET. Figure 7: The mechanistic models of G9a-dependent, gene-specific regulation of transcription. ( a ) c-Myc is a dual-functional transcription factor dependent upon either an acetyl-lysine or methyl-lysine-enriched environment when chronically active G9a promotes its transcriptional activity to repress select genes. ( b ) Chronically active G9a selectively recruits defined protein complexes into the chromatin of pro-inflammatory genes for their silencing during ET. Full size image Previous evidence from independent studies suggests that, in endotoxin-tolerant macrophages, nucleosomes are repositioned from permissive to repressive locations, and both promoter chromatin remodelling and NF-κB transactivation are disrupted [56] . Our repressome findings now provide the molecular illustration that the specificity of the inflammation-phenotypic chromatin reprogramming is controlled by particular transcription factors and co-factors that are selectively recruited: during ET, select transcriptional repressors including RelB, YY1, c-Myc were first recruited into the T-gene chromatin [17] , [57] to replace the transcriptional activators such as RelA/p65 ( Fig. 2f ), and then interact with the chronic-activated G9a which in turn stabilizes the binding of these factors to select classes of the genes. This idea is consistent with the previously reported correlation between RelB expression and the induction of repressive nucleosome positioning [58] as well as the in vitro interaction between GST-tagged G9a and RelB during ET [17] . Meanwhile, the major factor complexes associated with chromatin plasticity and mobilizations including NuRD and SWI/SNF complexes were simultaneously identified in the G9a repressome, indicating that chronic-active G9a interacts with these complexes to integrate activities of nucleosome positioning, ATP-dependent chromatin remodelling and transcriptional repressors. Also supported by comparative proteomic experiments on paired wild-type and G9a-KD macrophages, in which global protein products of G9a-silenced genes were identified, we concluded that chronic-active G9a participates in the co-regulation by select transcriptional repressors in cross talk that synergistically pronounce the gene-specific repression. On a systems view, we are the first to demonstrate that as the writer of the chromatin-repressive mark H3K9me2, in a methylation activity-dependent manner, G9a couples select biological pathways/programs across multi-phases of transcription including DNA binding, nucleosome localization and transcription factor recruitment to the gene-specific epigenetic regulation by recruiting specific complexes to the chromatin of T-genes, which systematically define a transcriptionally silenced chromatin ( Fig. 7b ). Technically, our ChaC approach can generate activity-based interactome data in a physiologically accurate manner and is generically applicable to dissect a variety of phenotypic chromatin architectures in the context of a functional protein complexome. Reagents and mice LPS ( Escherichia coli 0111:B4, ultrapure) was purchased from InvivoGen (USA, Invivogen, cat# tlrl-pelps). HEK 293 stable TLR4-MD2-CD14 cell line was also purchased from InvivoGen. All components of cell culture media and protease inhibitor cocktails were purchased from Sigma (St, Louis, MO). Fetal bovine serum was obtained from Gibco (Life Technologies). Trypsin was purchased from Promega (Madison, WI). All chemicals were either sequence or HPLC grade unless specifically indicated. Antibodies against G9a cat# 07-551 (1:1,000), H3K9me2 #07-441 (1:1,000), H3K4me3 #07-473 (1:1,000) and H3K4me2K9me2 #07-1843 (1:2,000) were purchased from Millipore. Antibodies for c-Myc (N-262) #sc-764x (1:2,000), Brg1 (H-88) #sc-10768x (1:2,000), HDAC1 #sc-7872 (1:1,000), MTA1 #sc-373765 (1:1,000), YY1 (H-414) #sc-1703 (1:1,000), SIRT-1 #sc-15404 (1:1,000) and β-Actin #sc-1616 (1:2,000) were from Santa Cruz. Antibodies for H3 #ab1791 (1:5,000), γ-Tubulin #ab11316 (1:5,000) were from Abcam. Antibodies for H3K36me2 #39255 (1:5,000) and H3K27me3 #39156 (1:5,000) were purchased from Active Motif; for H3K27me2 #PA5-17376 (1:2,000) was from PIERCE; for p-p65 (S536) #3033 (1:1,000) was from Cell Signaling; for NSD3 #GTX109396 (1:1,000) was from GeneTex; CtBP2 #612044 (1:2,000) was from BD Biosciences. Anti-HA (clone HA-7) (1:4,000) and anti-flag M2 (clone M2) (1:4,000) antibodies were from Sigma. Male or female mice (6–8 weeks old; C57BL/6 strain) were used. All mouse procedures in this study were approved by the Institutional Animal Care & Use Committee (IACUC) at the University of North Carolina at Chapel Hill. Uncropped immunoblots are provided in Supplementary Fig. 14 . BMDM culturing and AACT/SILAC labelling Bone marrow progenitors were rinsed out from femur and tibia bones of C57BL/6 wild-type mice. Red blood cells were removed by ACK Lysing Buffer (Gibco). Bone marrow cells were cultured on petri dishes for 6 days in the DMEM supplemented with 10% fetal bovine serum, 20% L929-conditioned media, either regular or AACT-containing media. On day 7, BMDMs were lifted with cold TEN buffer (40 mM Tris-HCl pH7.4, 1 mM EDTA, 150 mM NaCl) and replated on tissue-culture treated plates. Stable isotope labelling growth media were prepared [7] . In brief, the growth media in depletion of lysine and arginine were supplemented with either 13 C 6 -lysine (K6)/ 13 C 6 -arginine (R6) or 13 C 6 15 N 2 -arginine (K8)/ 13 C 6 15 N 4 -arginine (R10), respectively (Sigma-Aldrich cat#643459, cat#643440, cat#608041, cat#608033). Primary BMDMs or Raw264.7 cells were either left unstimulated (‘N’), or subjected to a single LPS stimulation at 1 μg ml −1 , or first primed with 100 ng ml −1 LPS to induce ET for 24 h (‘T’), followed by the second LPS challenge at 1 μg ml −1 (‘TL’). Cells were grown at 37 °C in a humidified atmosphere and 5% carbon dioxide in air. Histone sample preparation Core histone proteins were prepared by Histone Purification Mini Kit (Active Motif cat#40026). In brief, adhered cells were washed with prewarmed serum-free media twice and were then harvested. The pellet was lysed with 1.5 ml extraction buffer per 2 × 10 7 cells and homogenized by repetitive pipetting. The cell lysate was processed under agitation for 2 h at 4 °C before the crude histone was clarified, neutralized and loaded onto the column. Histone proteins were purified by a C8 column and were precipitated by 4% perchloric acid according to the manufacturer’s instructions and were resolved in HPLC water. All steps were processed on ice or in cold room, for the maximum preservation of histone modifications. HPLC purification of histone and top–down mass spectrometry Histone proteins were injected onto a C-8 column with a particle size of 7 μm and the inner diameter of 2.1 mm (Perkin Elmer cat# 07110060) using an Agilent 1100 series RP-HPLC (Agilent, Santa Clara CA). The core histone proteins were separated using the gradient: 35–60% acetonitrile/0.1%trifluoroacetic acid for 75 min. Protein elution was monitored by ultraviolet absorption at a wavelength of 214 nm. Histone fractions were collected, lyophilized and then subjected to μESI-FTICR-MS analysis [59] . We also explored the use of a LTQ Orbitrap Velos mass spectrometer (Thermo Scientific, San Jose, CA) to perform top–down MS analysis of inflammation-phenotypic HPLC-purified, full-length H3.1 (The methodology innovation will be reported elsewhere). In brief, mass analysis was achieved in both Full-MS, SIM of +19 charge state and electron transfer dissociation-tandem mass spectrometry modes [60] with an instrument resolution setting of 120,000 at m/z 400 Da. All samples were dissolved in a solution of 50:50 methanol:water and 1% formic acid and introduced to the mass spectrometer via direct infusion at a flow of 8 μl min −1 . ETD was performed specifically on the isotopic clusters of two peaks (average m/z of 809.29 Th and m/z of 810. 03 Th) for the +19 charge state that correspond to various isoforms showing abundance variations, respectively, under N, NL and TL states. The lower m/z range: 200–780 Th product ions were processed manually in all electron transfer dissociation-tandem mass spectrometry spectra by assigning sequence ions to theoretical masses corresponding to a diverse set of combinatorial PTMs [61] that includes R2(me2), R2(me), K4(ac), K4(me2), K4(me), K9(ac), K9(me2), K9(me), K9(me3), K14(ac), K14(me), K14(me2), K27(ac), K27(me), K27(me2), K36(ac), K36(me) and K36(me2). Nuclear extraction Nuclear extract was prepared [62] . In brief, BMDM cells were collected and resuspended in hypotonic buffer A (10 mM HEPES pH 7.9, 1.5 mM MgCl 2 , 10 mM KCl, 1 mM phenylmethylsulfonyl fluoride (PMSF), 1 mM DTT and protease inhibitor cocktail). After incubating for 10 min on ice, the swollen cell pellet was spun down and resuspended in two volumes of Buffer A and homogenized to release cytosolic fraction. Nuclei were collected by centrifugation at 14,000 r.p.m. for 10 min and homogenized with 10 strokes in Buffer C (20 mM HEPES pH 7.9, 1.5 mM MgCl 2 , 0.2 mM EDTA, 420 mM NaCl, 25% Glycerol, 1 mM PMSF, 1 mM DTT and protease inhibitor cocktail). Extraction was allowed to proceed under agitation for 30 min at 4 °C before the nuclear extract was clarified by centrifugation at 14,000 r.p.m. for 30 min at 4 °C. The extract was dialyzed overnight to 50 volumes buffer D (20 mM HEPES pH 7.9, 0.2 mM EDTA, 100 mM KCl, 20% Glycerol, 1 mM PMSF, 1 mM DTT and protease inhibitor cocktail). Adding Triton-X-100 to a final concentration of 0.1% and centrifuging again, the supernatant was the nuclear extract. Chromatin activity-based chemoproteomics An aminopropyl linker was added for coupling UNC0638 (ref. 26 ) to ECH sepharose 4B beads (General Electric cat# 17-0571-01). UNC0638 immobilized on sepharose beads were washed in Buffer D with 0.1% Triton-X-100 twice before addition into the nuclear extract. After incubation overnight, the beads were washed with 250 mM KCl buffer (20 mM HEPES pH 7.9, 0.2 mM EDTA, 250 mM KCl, 20% Glycerol, 1 mM PMSF, 1 mM DTT and protease inhibitor cocktail) five times. The pull-down products were eluted by boiling the beads in 2 × SDS–polyacrylamide gel electrophoresis loading buffer for 10 min. For histone peptide pull-down experiments, histone H3 N-tail peptides were synthesized with a biotin tag, then the peptide was conjugated to streptavidin beads and the pull-down experiment was carried out in a similar way as UNC0638 pull-down except for that the washing buffer was substituted by a low-stringent buffer containing 100 mM KCl. The pull-down products were resolved by SDS–polyacrylamide gel electrophoresis, either for immunoblotting or followed by in-gel tryptic digestion before MS analysis. Stable shRNA-mediated knockdown of G9a The lentiviral plasmids for the shRNA targeting mouse Ehmt2 (G9a) in a vector pLKO.1 were purchased from Thermo Scientific Open Biosystems. The shRNA-Ehmt2 target sequence is TTGTTATCTAAATCGAAGAGG . A pLKO.1 EV without shRNA sequence was used as the wild-type control. To generate virus, pLKO.1-shRNA plasmids were co-transfected into 293T cells with ViraPower Mix (Invitrogen) by jetPRIME in vitro DNA and short interfering RNA transfection reagent (Polyplus). Viral supernatants were collected 24 and 48 h following transfection and were used to transduce Raw264.7 cells by spinoculation. Forty-eight hours after the transfection, 8 μg ml −1 puromycin was added to initially select puromycin-resistant clones. The stable clones were maintained in the media containing 4 μg ml −1 puromycin. The level of G9a expression was examined for individual clones. Those clones with at least 90% knockdown efficiency were used in the experiments. Quantitative proteomic profiling protein expression during ET The pair of Raw264.7 cell lines either stably expressing shRNA for G9a KD, or the wild-type with EV were cultured for AACT labelling as described above. Both sets of the cells were primed with a low-dose LPS at 100 ng ml −1 for 24 h and then challenged with a high-dose LPS at 1 μg ml −1 to introduce ET. Cells were harvested 2 h after LPS challenge and lysed in buffer containing 8 M urea, 50 mM Tris-HCl pH 8.0, 75 mM NaCl, 1 mM MgCl 2 , 500 U Benzonase and protease inhibitor cocktail. Equal amounts (0.5 mg) of the lysate from each pool were mixed. The mixed protein pool was first reduced with DTT followed by cysteine alkylation with iodoacetamide, and then diluted fourfold by 25 mM Tris-HCl pH 8.0, 1 mM CaCl 2 . The diluted protein mixture was digested with trypsin (Promega #V5113) at 37 °C overnight and then replenished trypsin to further digestion for another 6 h. The peptides were desalted on Sep-Pak Light C18 cartridge (Waters, Milford, MA) and dried. The peptides were dissolved in 10 mM ammonium formate pH 10.0 and subjected to high-pH RPLC separation performed with an Xbridge C18, 250 × 4.6 mm column containing 5 μM particles and equipped with a 20 × 4.6 mm guard column (Waters, Milford, MA). The mobile-phase A consisted of 10 mM ammonium formate (pH 10.0) and B 10 mM ammonium formate (pH 10.0) with 90% acetonitrile. Peptide separation was accomplished using the following gradient: from 0 to 5% B in 5 min, from 5 to 35% B in 30 min, from 35 to 70% B in 7.5 min and held at 70% B for an additional 5 min. Sixty fractions were collected and concatenated into 30 fractions by combining fractions 1, 21, 41; 2, 22, 42. The samples were dried and desalted on StageTip containing 4 × 1 mm C18 extraction disk (3 M). Mass spectrometry analysis of ChaC pull-down products Peptide samples were dissolved in 0.1% formic acid and subjected to nanoLC-MS/MS analysis by using an online nanoLC ultra2D system (Eksigent) coupled to an LTQ Orbitrap Velos mass spectrometer (Thermo Scientific, San Jose, CA) [7] . In brief, LC-MS experiments were performed in a data-dependent mode with Full-MS (externally calibrated to a mass accuracy of <5 p.p.m. and a resolution of 60,000 at m/z 400) followed by CID MS/MS of the top 10 most intense ions. Mass spectra processing and peptide identification were performed on the Andromeda search engine in MaxQuant software (Ver. 1.2.0.18) (ref. 63 ) against a mouse UniProt database. All searches were carried out with cysteine carbamidomethylation as a fixed modification, while methionine oxidation and protein amino-terminal acetylation as dynamic modifications. Peptides were confidently identified using a target-decoy approach with a peptide false discovery rate (FDR) of 1% and a protein FDR of 1%. Data processing and statistical analysis were performed on Perseus (Version 1.2.0.17) (ref. 64 ). AACT/SILAC quantitation (3-plex K0R0, K6R6, K8R10 or 2-plex K0R0, K8R10) analysis was carried out similarly as previous described [7] . The AACT ratios of the proteins were derived from the comparison of the extracted ion chromatogram peak areas of all matched light (L) peptides with those of the medium (M) or heavy (H) peptides. The ratios of M/L or H/L were also verified by visual inspection of the raw mass spectra. Biological processes are categorized by DAVID ( http://david.abcc.ncifcrf.gov/ ). Protein–protein interaction network analysis was performed by an online bioinformatics tool STRING ( http://string-db.org ). TF regulatory network was preceded by IPA (Ingenuity pathway analysis). RNA preparation and quantitative PCR Total RNA was isolated using RNeasy kit (Qiagen). First-strand cDNA was synthesized by M-MLV reverse transcriptase (Promega, car# M170B) and diluted 10 times for quantitative PCR. Real-time PCR was performed using SYBR Green Master Mix (Thermo Fisher, cat# 0221). All measurements were normalized to GAPDH and represented as relative ratios. PCR primers for real-time PCR are summarized in Supplementary Table 5 . Sample collection of the macrophage secretome Primary BMDM cells were primed with 250 nM UNC0638 or DMSO for 16 h. Cells were then either left unstimulated (‘N’) or subjected to a single LPS challenge at 500 ng ml −1 for indicated hours (‘NL’) or first primed with 100 ng ml −1 LPS to induce the ET for 24 h, followed by the second LPS challenge at 500 ng ml −1 for indicated hours (‘TL’). Before the LPS challenge, cells were washed once and cultured in serum-free DMEM without phenolred, containing 1 mM sodium pyruvate and 10 mM L -glutamine. The secreted proteins were harvested and prepared [51] . Label-free quantitative analysis of macrophage secretome LFQ secretome analyses were performed via reversed phase LC-MS/MS using a Proxeon 1000 nano LC system coupled to an Q Exactive mass spectrometer (Thermo Scientific, San Jose, CA). The Proxeon system was configured to trap peptides using a 3-cm long 100 μm i.d. C18 column at 5 μl min −1 liquid flow that was diverted from the analytical column via a vent valve, while elution was performed by switching the valve to make the trap column in line with a 15-cm long, 75 μm i.d., 3.5 μm, 300-Å particle; C18 analytical column. Analytical separation of all the tryptic peptides was achieved with a linear gradient of 2–35% buffer B over either 240 min at a 300 nl min −1 flow rate, where buffer A is aqueous solution of 0.1% formic acid and buffer B is a solution of acetonitrile in 0.1% formic acid. LC-MS experiments were also performed in a data-dependent mode with Full-MS (externally calibrated to a mass accuracy of <5 p.p.m. and a resolution of 70,000 at m/z 200) followed by HCD-MS/MS of the top 20 most intense ions. High-energy collision-activated dissociation (HCD)-MS/MS was used to dissociate peptides at normalized collision energy of 27 eV in the presence of nitrogen bath gas atoms. All secretome samples consisting of three biological replicates were subjected to single-shot independent LC-MS runs resulting in the production of 48 LC-MS runs for global peptide analysis. Mass spectra were processed and peptide identification was performed using Andromeda search engine found in MaxQuant software ver. 2.2.1. (Max Planck Institute, Germany) All protein database searches were performed against the UniProt mouse protein sequence database. Peptides were identified with a target-decoy approach using a combined database consisting of reverse protein sequences UniProt mouse sequence and common repository of adventitious proteins (cRAP). The cRAP database was obtained from the Global Proteome Machine ftp site ( ftp://ftp.thegpm.org/fasta/cRAP ). Peptide identification was made with a FDR of 1% while peptides were assigned to proteins with a protein FDR of 5%. A precursor ion mass tolerance of 20 p.p.m. was used for the first search that allowed for m/z retention time recalibration of precursor ions that were then subjected to a main search using a precursor ion mass tolerance of 5 p.p.m. and a product ion mass tolerance of 0.5 Da. Search parameters included up to two missed cleavages at KR on the sequence and oxidation of methionine as a dynamic modification. All protein and peptide identifications are reported by filtering for reverse and contaminant proteins. Label-free quantitation was based on the peak area [65] , [66] , [67] . The measured area under the curve of m/z and retention time aligned extracted ion chromatogram (XIC) of a peptide was performed via the label-free quantitation module found in MaxQuant (ver. 1.3.0.5) (ref. 65 ). All replicates (biological and technical replicates) of each experimental conditions: N, NL-16 h, TL-16 h, were included in the LFQ experimental design with protein-level quantitation and normalization performed using unique and razor peptide features corresponding to identifications filtered with a peptide FDR of 0.01 and protein FDR of 0.05. The MaxQuant protein groups and evidence files were processed using the statistical analysis and visualization features found in Perseus (ver. 1.4.1.3) (Max Planck Institute, Germany) Tagged immunoprecipitation HEK 293 stable TLR4-MD2-CD14 cell line (Invivogen) was transfected with indicated constructs by jetPRIME transfection reagent (Polyplus, cat#114–15). The cells were harvested from indicated conditions and lysed with RIPA buffer containing 20 mM Tris-HCl, 137 mM NaCl, 2 mM EDTA, 10% glycerol, 0.5% NP-40 and 1 mM PMSF. Cell lysates were incubated with affinity beads for overnight at 4 °C on rotator. Affinity beads were washed with RIPA buffer four times before subjected to immunoblot assay. Chromatin immunoprecipitation ChIP experiments for studying histone modifiers and TFs were carried out in dual crosslinking way [68] with minor modifications. Cells were fixed using 2 mM DSG (disuccinimidyl glutarate, ProteomChem #c1104) for 45 min. Formaldehyde (1% v/v) was then added and incubated for 15 min. Crosslinking reactions were quenched by adding glycine to 0.1 M, followed by PBS washing. Cells were scraped and nuclei were pelleted by 0.5% NP-40 lysis buffer (50 mM pH 8.0 Tris-HCl, 85 mM KCl, 0.5% NP-40). The nuclear fraction was extracted with RIPA buffer (50 mM pH 8.0 Tris-HCl, 150 mM NaCl, 1 mM EDTA, 1% Triton-X-100, 0.1% SDS, 0.1% sodium deoxycholate) and sonicated to 200–1,000 bp DNA fragments, then incubated overnight with the antibody. The antibody complexes were linked to protein A/salmon sperm DNA beads (Cell Signaling, cat #9007) and washed thoroughly. The complexes were then eluted from the beads by 1% SDS, and incubated with NaCl to reverse the crosslinked products. Later, proteins were digested by protease-K and the released DNA was purified by QIAquick PCR purification Kit (Qiagen, cat #28104), and processed to quantitative PCR assay. ChIP experiments for studying histone post-PTMs were started from a one-step fixation of 1% (v/v) formaldehyde for 10 min, followed by the same steps as dual crosslinking ChIP described above. PCR primers for real-time PCR are summarized in Supplementary Table 6 . ChIP-seq ChIP experiments against c-Myc antibody (Santa Cruz cat#sc-764x) were processed in G9a KD stable cell line and wild-type control Raw264.7 cells, respectively, following the one-step formaldehyde fixation procedure. ChIP’s DNA from two cell lines and INPUT from wild-type cells were subjected to library construction using ThruPLEX-FD Prep Kit (RUBICON GENOMICS, cat# R40012-08). DNA libraries are cleaned up with Agencourt AMPure XP beads (Beckman Coulter cat# A63880), quantified by Qubit 2.0 fluoremeter and qualified by Experion automated electrophoresis system (BIO-RAD). Three libraries were pooled and subjected to deep sequencing on Illumina Hiseq 2000. ChIP-seq data were aligned using Bowtie 2 (Version 2.1.0) (ref. 69 ) to build version NCBI37/mm9 of mouse genome. ChIP-seq-enriched regions over INPUT background were identified with the peak finding algorithm of MACS [70] (Model based analysis of ChIP-seq). G9a activity assay 293/TLR4-MD2-CD14 cells were transfected with tagged G9a plasmids and tagged-c-Myc plasmids as indicated. The next day, the transfected cells were primed with 100 ng ml −1 LPS for 24 h and then challenged with 1 μg ml −1 LPS for another 45 min. Cells were harvested and subjected to tagged IP with anti-flag affinity beads. After overnight incubation, anti-flag beads were washed with reaction buffer (Tris-HCl 20 mM pH 8.0, 25 mM NaCl, 0.025% Tween-20 and 1 mM DTT). In vitro assay was carried out as previous described [26] . In brief, anti-flag beads were incubated with 5 μM S -adenosyl methionine and 2 nM fluorescent labelled H3 N-tail peptides (ARTK 4 (me)QTARK 9 STGGK 14 -(5-FAM)) in reaction buffer. After incubation for 2 h at 25 °C, 40 pg μl −1 endoproteinase-LysC (Endo-LysC) was added and allowed to digest the remaining unmethylated substrate peptides for 1 h before separation on the Caliper LabChIP EZ Reader II (Caliper Life Sciences, Hopkinton, MA). The histone H3 lysine 9 methyltransferase activity was represented as the percentile of peptide substrate being methylated. Recombinant G9a was applied as the positive control. The reactions lacking catalytic enzyme or methyl donor S -adenosyl methionine were applied as negative controls. NF-κB reporter assay 293/TLR4-MD2-CD14 cells were seeded on 24-well plates 1 day before transfection so that they will be 90% confluent at the time of transfection. The next day, the cells were transfected with 225 ng pGL2-ELAM promoter Firefly luciferase transgene plasmid and 450 ng plasmids indicated. The pRL-TK plasmid, which expresses Renilla luciferase, was transfected into cells at 75 ng as an internal control to normalize transfection efficiency and sample handling. The cells were stimulated with 1 μg ml −1 LPS for 6 h before harvesting. The activities of the two kinds of luciferase were measured with their respective substrates with a dual luciferase assay kit (Promega). The luminescence reads reflecting NF-κB activity were obtained from the division of Firefly luciferase reads by Renilla luciferase reads. The data represented in the corresponding figures were the luminescence normalized to the control sample transfected with EV instead of functional plasmids. y axis indicates relative NF-κB activity. The error bar represents the s.d. of triplicates. Similar results were obtained in three independent biological experiments. Measurements of c-Myc stability and degradation Raw264.7 or TLR4/MD2/CD14 293 cell lines were primed with 100 ng ml −1 LPS for 24 h and then treated with 1 μg ml −1 cycloheximide (Sigma-Aldrich #C4859) for indicated time. Cells were harvested and subjected to immunoblot analysis by using anti-c-Myc antibody. Exposed films of immunoblot were scanned and quantified by ImageJ densitometry software. The intensity of each band was plotted in scatter plot and c-Myc half-life was determined on computed curve. Raw264.7 cells were primed with 100 ng ml −1 LPS for 24 h and then treated with 10 μM MG-132 for time indicated. C-Myc accumulation was reflected in immunoblot against c-Myc by short- and long-exposure. β-Actin and γ-Tubulin were represented as loading controls. Clonogenic survival assay Raw264.7 cells were counted and plated in six-well cell culture plates with 50, 100 and 200 viable cells in duplicated wells. Cells were primed with 100 ng ml −1 LPS for 48 h to reach the condition of ET and replenished with fresh media. UNC0638 (1 μM) was replenished into the media. After 9-day cell growth, cell colonies were washed with PBS, fixed with a mixture of methanol-acetic acid (3:1 in volume ratio) for 10 min, stained with 10% Giemsa (Ricca) for 30 min, gently washed with water and air dried. The colonies containing more than 20 cells were counted and the percentage of the survived cells under each condition was determined compared with the number of colonies on non-LPS or UNC0638-treated plates. How to cite this article: Liu, C. et al . A chromatin activity-based chemoproteomic approach reveals a transcriptional repressome for gene-specific silencing. Nat. Commun. 5:5733 doi: 10.1038/ncomms6733 (2014).